Nanoscale chromatin profiling of gastric adenocarcinoma reveals cancer-associated cryptic promoters and somatically acquired regulatory elements Chromatin alterations are fundamental hallmarks of cancer. To study chromatin alterations in primary gastric adenocarcinomas, we perform nanoscale chromatin immunoprecipitation sequencing of multiple histone modifications in five gastric cancers and matched normal tissues. We identify hundreds of somatically altered promoters and predicted enhancers. Many cancer-associated promoters localize to genomic sites lacking previously annotated transcription start sites (cryptic promoters), driving expression of nearby genes involved in gastrointestinal cancer, embryonic development and tissue specification. Cancer-associated promoters overlap with embryonic stem cell regions targeted by polycomb repressive complex 2, exhibiting promoter bivalency and DNA methylation loss. We identify somatically acquired elements exhibiting germline allelic biases and non-coding somatic mutations creating new promoters. Our findings demonstrate the feasibility of profiling chromatin from solid tumours with limited tissue to identify regulatory elements, transcriptional patterns and regulatory genetic variants associated with cancer. Gastric cancer (GC) is a major cause of global cancer mortality [1] . Most GCs are adenocarcinomas, and recent exome- and whole-genome sequencing studies have revealed new GC driver genes and mutational signatures [2] , [3] , [4] . Besides protein-coding genes, somatic changes in regulatory elements located in non-coding genomic regions are also likely contributors to malignancy, as these elements can profoundly influence chromatin structure and gene expression [5] , [6] , [7] . Regulatory elements can be altered by epigenetic mechanisms including changes in DNA and histone methylation patterns—in many cancers, these have been associated with methylation-induced transcriptional silencing of tumour suppressor genes [8] , chromosomal instability [9] and loss of imprinting [10] . In GC specifically, several studies have supported a major role for epigenetic alterations in gastric tumorigenesis. For instance, infection by Helicobacter pylori , a type I GC carcinogen, has been shown to induce aberrant DNA methylation patterns in normal stomach mucosa [11] . Tumour suppressor genes such as CDH1 and RUNX3 are often silenced in primary GCs by promoter DNA methylation [12] , [13] , and changes in DNA methylation have also been associated with GC prognosis, chemosensitivity and drug resistance [14] , [15] , [16] . More recently, genome-wide studies have highlighted a role for both global and non-CpG island methylation in specific GC subtypes [17] , [18] , [19] , and exome-sequencing studies have revealed that genes involved in chromatin modification such as ARID1A are frequently mutated in GC [2] , [4] . Currently however, the vast majority of epigenetic studies in GC have focused on characterizing patterns of aberrant DNA methylation. In contrast, few studies have explored on a genomic scale the repertoire of histone modifications (‘chromatin marks’), and their associated regulatory elements, that are somatically altered during gastric carcinogenesis [20] . Regulatory elements associated with specific histone modifications and chromatin marks include promoters and enhancers. To date, most histone modification/chromatin mark studies in cancer have used immortalized cell lines, since existing protocols require significant amounts of biological material [6] . However, cancer lines cultured in vitro can display epigenetic patterns distinct from primary tumours [21] , and cell lines may also undergo in vitro adaption, acquiring genetic and epigenetic changes due to extensive passaging [22] . Identification of somatically acquired alterations using cancer cell lines is also difficult, as they often lack matched normal counterparts. To address these limitations, we apply in this study nanoscale chromatin profiling (Nano-chromatin immunoprecipitation (ChIP)-seq) to measure multiple chromatin marks in primary gastric adenocarcinomas and matched normal gastric tissues. Nano-ChIP-seq is a recently described microscale chromatin profiling technique validated down to the 1,000-cell scale [23] . By comparing the chromatin profiles of malignant tissues with their matched non-malignant counterparts, we identify hundreds of somatically altered promoters and predicted enhancers. Interestingly, when compared against reference transcript databases (for example, RefSeq), a significant proportion of the somatically acquired promoters localize to regions outside standard promoter annotations (‘cryptic promoters’) and are frequently associated with expression of non-canonical transcripts with altered 5′ exons. Integration with ENCODE data reveals that cancer-associated promoters frequently overlap with genomic regions targeted by PRC2 (polycomb repressive complex 2) in embryonic stem cells (ESCs). Finally, we survey genetic variation in the somatically altered regulatory elements and identify candidate germline variants and somatic mutations influencing gene regulation. Taken collectively, our findings demonstrate the feasibility of profiling chromatin from solid tumours with limited tissue and highlight a pervasive and unexpected role for cryptic promoters in the reactivation of gene expression programs in GC. Our results also suggest the potential utility of cryptic promoters as biomarkers of gastric malignancy. Nano-ChIP-seq chromatin profiling of primary gastric tumours We profiled five matched pairs of primary GCs and normal gastric samples using Nano-ChIP-seq [23] ( Supplementary Fig. 1 , Fig. 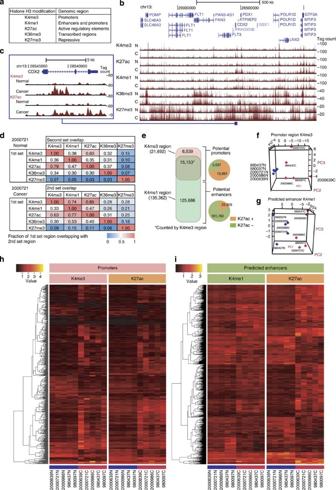Figure 1: Nano-ChIP-seq chromatin profiles of primary gastric adenocarcinomas. (a) Chromatin marks analysed. (b) Chromatin profile of GC 2000721 and matched normal gastric tissue (C and N, respectively). Shown is a representative UCSC Genome Browser display of theCDX2gene locus and adjacent genes. RefSeq transcripts and histone modifications are displayed. (c) Close-up view of theCDX2gene, demonstrating K4me3 and K27ac gain in GC. (d) Chromatin mark peak overlaps in normal (top) and GC (bottom). GC 2000721 is depicted. Numbers represent the fraction of first set regions (vertical) overlapping with second set regions (horizontal). Blue=exclusive, red=overlapping. (e) GC predicted enhancers and promoters. Promoter and predicted enhancer regions were further classified by their overlap with K27ac signals (right circles). (f,g) PCA plots of normal (blue) and GC (red) samples based on somatically altered (f) promoter (K4me3) and (g) predicted enhancer (K4me1) regions. The top three principal components were used. See Methods for statistical criteria used to define the promoter and enhancer subsets. (h,i) Clustering heatmaps of normal (blue) and GC (red) samples based on somatically altered (h) promoter and (i) predicted enhancer (K4me1) regions. K27ac patterns are also shown. Color intensities correspond to normalized RPKM values. 1a , Supplementary Table 1 for clinical details). The chromatin marks included (i) tri-methylated histone H3 lysine 36 (K36me3), associated with transcribed regions; (ii) tri-methylated histone H3 lysine 27 (K27me3), repressed regions; and (iii) histone H3 K4me3, K4me1 and K27ac (ac=acetylation), marking active promoters and predicted enhancers [24] , [25] , [26] . For each mark, we generated >45 million uniquely mapped Illumina sequencing tags and called peak regions using CCAT ( Supplementary Fig. 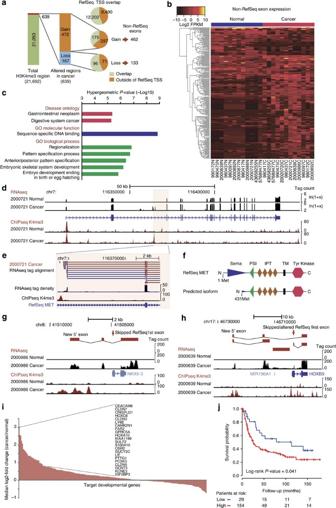Figure 2: Cancer-associated promoters in GC. (a) Cancer-associated promoters are frequently associated with non-RefSeq TSSs (‘cryptic promoters’). Cryptic promoter proportions associated with all promoters (‘total’) and promoters lost in cancer (‘loss’) are provided as references. Cancer-associated promoters are also associated with expressed non-RefSeq transcripts from RNAseq data (right most numbers). (b) Heatmap showing expression status of non-RefSeq transcripts exhibiting greater than fourfold expression changes between normal tissues and gastric tumours (FPKM). The transcripts are associated with 192 cancer-associated promoters. (c) GREAT analysis demonstrating enriched gene categories for cancer-associated promoters. All enriched terms withP<6 × 10−6from the original GREAT34output are listed. (d,e) Cryptic promoter-drivenMETexpression. RNAseq and K4me3 tracks are shown. (e) Close-up view of the cryptic promoter region. Mapped RNAseq reads that span exon junctions are connected with lines (forward read in blue, reverse read in red), showing representative ‘split’ RNAseq reads confirming linkage of the promoter to downstreamMETexons. (f) MET functional domains. The predicted cryptic promoter-driven transcript encodes an N-terminal truncated protein lacking the Sema domain. (g) Cryptic promoter-drivenNKX6-3expression. RNAseq and K4me3 tracks are shown. RNAseq alignments are provided inSupplementary Fig. 13. (h) Cryptic promoter-drivenHOXB9expression. RNAseq alignments are provided inSupplementary Fig. 14. (i) Expression levels of K4me3-marked genes between GCs (n=185) and matched normals (n=89). A significant proportion of genes are upregulated in GC (upregulated genes=143; total target genes=218; one sample proportion testP-value=5.68 × 10−6). (j) Survival analysis comparing patient groups with GCs exhibiting high and low expression of genes driven by cancer-associated promoters. Kaplan–Meier survival analysis of clusters within the Singaporean cohort (totaln=183) with ‘high’ (n=154) and ‘low’ (n=29) enrichment of the target gene signature. The signature is prognostic in this cohort (P=0.04, log-rank test)), with worse prognosis observed for higher enrichment of the signature (hazard ratio (95% CI): 1.78 (1.02–3.13); Cox regressionP-value=0.044). 2 , Supplementary Table 2 ) [27] . Genomic regions in tumour samples exhibiting an abnormal abundance of ChIP input tags, likely reflecting genomic amplification, were excluded from downstream analyses ( Supplementary Fig. 3 ) [28] . We successfully obtained genome-wide chromatin profiles for both normal and cancer tissues ( Fig. 1b ), despite limited material (~5 mg tissue for all marks). For example, we observed cancer-specific gain of promoter activity (increased K4me3 and K27ac) at the CDX2 gene, associated with intestinal metaplasia [29] ( Fig. 1c ). Figure 1: Nano-ChIP-seq chromatin profiles of primary gastric adenocarcinomas. ( a ) Chromatin marks analysed. ( b ) Chromatin profile of GC 2000721 and matched normal gastric tissue (C and N, respectively). Shown is a representative UCSC Genome Browser display of the CDX2 gene locus and adjacent genes. RefSeq transcripts and histone modifications are displayed. ( c ) Close-up view of the CDX2 gene, demonstrating K4me3 and K27ac gain in GC. ( d ) Chromatin mark peak overlaps in normal (top) and GC (bottom). GC 2000721 is depicted. Numbers represent the fraction of first set regions (vertical) overlapping with second set regions (horizontal). Blue=exclusive, red=overlapping. ( e ) GC predicted enhancers and promoters. Promoter and predicted enhancer regions were further classified by their overlap with K27ac signals (right circles). ( f , g ) PCA plots of normal (blue) and GC (red) samples based on somatically altered ( f ) promoter (K4me3) and ( g ) predicted enhancer (K4me1) regions. The top three principal components were used. See Methods for statistical criteria used to define the promoter and enhancer subsets. ( h , i ) Clustering heatmaps of normal (blue) and GC (red) samples based on somatically altered ( h ) promoter and ( i ) predicted enhancer (K4me1) regions. K27ac patterns are also shown. Color intensities correspond to normalized RPKM values. Full size image Comparison of the chromatin marks revealed that regions of active transcription (K36me3) were exclusive to regions of repressive chromatin (K27me3) ( Fig. 1b,d , GC 2000721; see Supplementary Fig. 4 ). By merging K4me3 peak regions from the five tissue pairs, we predicted >21 K putative promoters marked by K4me3 ( Fig. 1e ). To predict potential enhancers, we then focused on those regions marked by K4me1 but not K4me3. Notably, the use of histone marks to accurately predict enhancers should still be regarded as work in evolution [25] , [30] , [31] , and in this study, technical assessment of our enhancer prediction method using ENCODE data [32] suggests a sensitivity and specificity range of 37–67% depending on cell line ( Supplementary Fig. 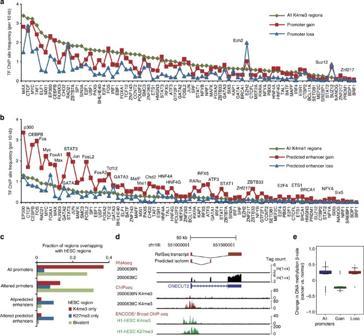Figure 3: Binding site analysis of cancer-associated regulatory elements. (a) Frequency of ENCODE-defined TFBSs overlapping with cancer-associated promoters (gained and lost). Values are presented as the number of TFBS per 10 kb coverage. TFs were sorted according to their frequency in all K4me3-defined promoter sets. EZH2, SUZ12 and ZNF217 binding sites are enriched (P<0.05, one-tailed Fisher’s exact test). The complete TF list is presented asSupplementary Fig. 17andSupplementary Table 7. (b) TFBS frequency in cancer-associated predicted enhancer regions. (c) Overlap analysis between ESC-defined univalent (K4me3 only, K27me3 only) or bivalent (K4me3 and K27me3) regions and GC promoters (all and cancer-associated) and GC-predicted enhancers (all and cancer-associated). Cancer-associated GC promoters exhibit an elevated proportion of bivalent regions, exceeding univalent regions (P<2.2 × 10−16, one-tailed Fisher’s exact test). (d) Genome browser view of theONECUT2locus as a representative cancer-associated promoter overlapping with an ESC-defined bivalent region. (e) Box plot depicting changes in DNA methylation β-values in all promoters and cancer-associated promoters (gained or lost).P-values (Wilcoxon test) are:P=7 × 10−48(all promoters versus gained promoters);P=0.48 (all promoters versus lost promoters);P=5.37 × 10−41(gained promoters versus lost promoters). 5 , Supplementary Table 3 ). As such, our set of potential enhancers should be regarded as ‘predicted enhancers’ instead of strictly true enhancers, and are referred to as such for the remainder on this report. Using this criteria, we identified >125 K predicted enhancers ( Fig. 1e ). Sixty-four percent of promoters were active (K27ac positive) and 19% of predicted enhancers were marked by K27ac in at least in one tissue ( Fig. 1e ). Identification of somatically altered regulatory elements To identify somatically altered promoters and potential enhancers in GC, we quantified and compared sequencing tag densities (read per kilobase per million tags, RPKM; see Methods) between GCs and normal tissues ( Fig. 1b , Supplementary Fig. 6 ). We identified 639 promoters exhibiting differential K4me3 and K27ac modifications between GCs and normal tissues, and 975 somatically altered predicted enhancers (see Methods). We independently validated by quantitative PCR (qPCR) 18 histone peaks (9 K27ac, 9 K4me3) exhibiting differences between GCs and normal tissues ( Supplementary Fig. 7 ; Pearson’s R =0.77–0.88 between Nano-ChIP-seq and qPCR values; P =0.015–0.001, two tailed Student’s t -test). Principal components analysis (PCA) and clustering analysis using these somatically altered elements confirmed a separation between GCs and matched normal tissues ( Fig. 1f–i , Supplementary Fig. 8 ). Of the somatically altered promoters, 270 could be associated with a nearby altered predicted enhancer (±500 kb [33] ). Of these, 81% ( n =219) of the promoter/predicted enhancer pairs showed concordant alterations (average promoter/predicted enhancer distance 166 kb, s.d. 145 kb). Reciprocally, of 975 altered predicted enhancers, 321 (33%) were associated with at least one altered promoter (within 500 kb), and of these 81% (261/321) of the predicted enhancer/promoter pairs showed concordant deregulation. These results suggest a strong and potentially functional link between somatic alterations in promoters and associated predicted enhancers in GC. Cryptic promoters and non-canonical mRNA transcripts We focused on the cancer-associated promoters. Gains of new promoters in primary GCs outweighed promoter losses (472 gained versus 167 lost, Fig. 2a ). Unexpectedly, the majority of gained promoters (58%) localized to regions >500 base pairs (bp) from annotated transcription start sites (TSSs) found in RefSeq, a reference database of transcript sequences. The fraction of ‘cryptic promoters’ in gained promoters was significantly greater than either the global promoter population or promoters lost in GC (~44%, P <7.1 × 10 −6 , Fisher’s exact test). 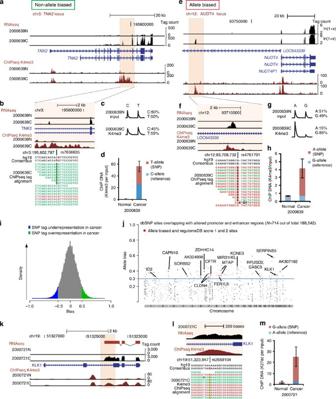Figure 4: Allele-specific regulatory elements associated with GC. (a–d) Non-allele biased and (e–h) allele-biased regulatory elements. (a,b) Genome browser view ofTNK2locus showing RNAseq and K4me3 tracks. (b) Close-up visualization of K4me3 sequence tags and SNPs. A comparable proportion of reference (C) and rs7636635 (T) SNPs are observed in K4me3-enriched sequence reads. (c) Genotyping of normal tissue confirms equivalent allele heterozygosity in normal tissues and K4me3-enriched sequence tags from tumours. (d) qPCR pyrosequencing confirms lack of K4me3 signal in normal tissue, and equal proportion of reference (C) and rs7636635 (T) allele K4me3-enriched sequence reads from tumours. Error bars are s.e.m. of qPCR signal (n=3). (e,f) Genome browser view ofNUDT4locus showing RNAseq and K4me3 tracks. (f) Close-up visualization of K4me3 sequence tags and SNPs. A bias favoring a higher proportion of rs4761701 SNP (A) over the reference allele (G) is observed. (g) Genotyping of normal tissue confirms equivalent allele heterozygosity in normal tissues but a bias towards rs4761701 SNP (A) in K4me3 sequence tags from tumours. (h) qPCR pyrosequencing confirms minimal K4me3 signal in normal tissue, and an rs4761701 SNP-biased proportion of sequence tags over the reference allele in K4me3 signals from tumours. Error bars are s.e.m. of qPCR signal (n=3). (i) Allele bias distribution across samples. Over- and underrepresentation of SNP tags in tumor tissues are marked in green and blue. (j) dbSNP sites mapping to altered regulatory regions. SNP sites are ordered following their chromosomal position (xaxis), and allele bias levels (yaxis). SNPs exhibiting allele bias (above blue horizontal line) and also predicted to affect protein binding based on RegulomeDB are marked in red. (k,l) Genome browser view of theKLK1locus showing RNAseq and K4me3 tracks. (l) Close-up view of K4me3 sequence tags and SNPs. A bias favoring a higher proportion of the known eQTL SNP rs2659104 (G) over the reference allele (A) is observed. (m) qPCR pyrosequencing confirms minimal K4me3 signal in normal tissue, and rs2659104 SNP-biased proportions of sequence tags over the parental allele in K4me3 signals from tumours. Error bars are s.e.m. of qPCR signal (n=3). Subsequent comparisons of the cancer-associated promoters to GENCODE and ENSEMBL, two other major transcript databases, also supported a large proportion of cryptic promoters (~40%; Supplementary Table 4 ). When compared against Nano-ChIP-seq data of four epithelial-derived GC cell lines, 67.7% of the 368 cryptic promoters were also present in the cell lines, suggesting that the majority of cryptic promoters are likely to occur in the epithelial cancer cells and not stromal-derived tumour components ( Supplementary Fig. 9 ). To ask if cancer-associated promoters (including cryptic promoters) were associated with bona fide RNA transcripts, we then performed RNA-sequencing (RNAseq) on 12 tumour/normal pairs, including the index 5 GCs. The majority of promoters (59.5%, 380 promoters) were associated with detectible RNA transcripts ( Fig. 2a ). We identified 192 transcripts exhibiting greater than fourfold expression changes in GCs compared with normal tissues, and almost half of these (48%, 92 promoters) were due to cryptic promoters, supporting their cancer-specific nature ( Fig. 2b ). Using targeted qPCR, we experimentally validated 10 cryptic promoter-associated transcripts ( Supplementary Fig. 10 ). Figure 2: Cancer-associated promoters in GC. ( a ) Cancer-associated promoters are frequently associated with non-RefSeq TSSs (‘cryptic promoters’). Cryptic promoter proportions associated with all promoters (‘total’) and promoters lost in cancer (‘loss’) are provided as references. Cancer-associated promoters are also associated with expressed non-RefSeq transcripts from RNAseq data (right most numbers). ( b ) Heatmap showing expression status of non-RefSeq transcripts exhibiting greater than fourfold expression changes between normal tissues and gastric tumours (FPKM). The transcripts are associated with 192 cancer-associated promoters. ( c ) GREAT analysis demonstrating enriched gene categories for cancer-associated promoters. All enriched terms with P <6 × 10 −6 from the original GREAT [34] output are listed. ( d , e ) Cryptic promoter-driven MET expression. RNAseq and K4me3 tracks are shown. ( e ) Close-up view of the cryptic promoter region. Mapped RNAseq reads that span exon junctions are connected with lines (forward read in blue, reverse read in red), showing representative ‘split’ RNAseq reads confirming linkage of the promoter to downstream MET exons. ( f ) MET functional domains. The predicted cryptic promoter-driven transcript encodes an N-terminal truncated protein lacking the Sema domain. ( g ) Cryptic promoter-driven NKX6-3 expression. RNAseq and K4me3 tracks are shown. RNAseq alignments are provided in Supplementary Fig. 13 . ( h ) Cryptic promoter-driven HOXB9 expression. RNAseq alignments are provided in Supplementary Fig. 14 . ( i ) Expression levels of K4me3-marked genes between GCs ( n =185) and matched normals ( n =89). A significant proportion of genes are upregulated in GC (upregulated genes=143; total target genes=218; one sample proportion test P -value=5.68 × 10 −6 ). ( j ) Survival analysis comparing patient groups with GCs exhibiting high and low expression of genes driven by cancer-associated promoters. Kaplan–Meier survival analysis of clusters within the Singaporean cohort (total n =183) with ‘high’ ( n =154) and ‘low’ ( n =29) enrichment of the target gene signature. The signature is prognostic in this cohort ( P =0.04, log-rank test)), with worse prognosis observed for higher enrichment of the signature (hazard ratio (95% CI): 1.78 (1.02–3.13); Cox regression P -value=0.044). Full size image Genes located near cancer-associated promoters were significantly enriched in gene sets related to gastrointestinal neoplasms/digestive system cancers ( Fig. 2c ; P <1 × 10 −5 by GREAT analysis [34] ). By analysing RNAseq sequence reads mapping to both the cryptic promoter-associated transcript and downstream RefSeq annotated transcript exons (otherwise known as ‘bridging’ or ‘split’ RNAseq reads), we discovered that cryptic promoters frequently drove expression of these nearby genes, through non-canonical messenger RNA (mRNA) isoforms with altered 5′ structures. For example, GC 2000721 exhibited tumour-specific expression of the MET receptor via an internal cryptic promoter ( Fig. 2d–f , Supplementary Fig. 11 ), producing a truncated isoform lacking the amino-terminal Sema domain, which regulates receptor dimerization and signalling [35] . 5′ RACE (rapid amplification of cDNA ends) analysis of MET -expressing Hs746T GC cells confirmed expression of this truncated MET isoform ( Supplementary Fig. 11 ). Western blotting analysis of NUGC4 GC cells, also predicted to express the truncated MET isoform, revealed expression of a shortened 100 kDa Met protein as well as the RefSeq-associated full length 190 kDa MET receptor. In contrast, only the full-length Met protein was observed in KATOIII GC cells that predominantly express the RefSeq-associated MET transcript ( Supplementary Figs 11 and 12 ). These results suggest that at least in the case of MET , aberrant mRNA transcripts driven by cryptic promoters may also be associated with aberrant proteins. Interestingly, genes located near cancer-associated promoters also exhibited significant functional enrichments in transcription factor function, embryonic development and cell-type specification ( P <2 × 10 −6 , false discovery rate (FDR), q <1 × 10 −3 by GREAT analysis; Fig. 2c ). For example, NKX6-3 , a nervous system and stomach tissue developmental regulator [36] , [37] , exhibited cancer-specific expression via a new 5′ exon skipping the canonical RefSeq NKX6.3 first exon ( Fig. 2g , Supplementary Fig. 13 ), resulting in a novel 184 amino acid N terminus modifying the homeobox domain ( Supplementary Fig. 13 ). Using RACE, we confirmed expression of these new 5′ exons in GC lines ( Supplementary Fig. 13 ). Similar altered 5′ transcript structures were also observed for the homeobox transcription factor HOXB9 [38] ( Fig. 2h , Supplementary Fig. 14 ). These results demonstrate cryptic promoter activation in GC. We note that in this study, the term ‘cryptic’ pertains specifically with respect to RefSeq, GENCODE and ENSEMBL, three major transcript databases used by the biomedical community. Since it is difficult, if not impossible, to comprehensively examine every transcript database in the literature, we cannot rule out that some of these cryptic promoters may be annotated in other databases. Nevertheless, our findings suggest that a significant number of cancer-associated promoters may produce non-canonical transcript isoforms, which in turn may generate proteins with altered structures and functions. To validate these expression patterns, we then confirmed that genes driven by K4me3-marked cancer-associated promoters exhibited similar tumour upregulation in an expanded microarray cohort of 185 GCs and 89 normal gastric tissues ( P =5.68 × 10 −6 , χ 2 test of proportions; Fig. 2i , Supplementary Fig. 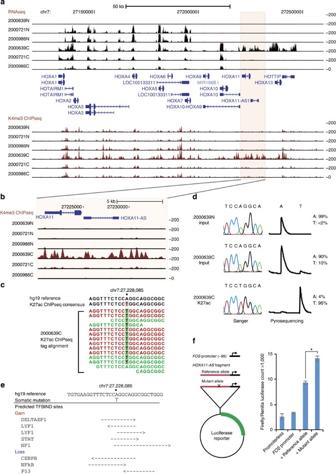Figure 5: Somatic regulatory mutations in GC. (a) Genome browser view of theHOXAlocus. (top) RNAseq data.HOXAgenes distal to (and including)HOXA11are expressed in GC 2000639 in a cancer-specific fashion. (Bottom) K4me3 signals confirm an altered chromatin domain in this region. (b) Close-up view of theHOXA11region. Cancer-specific acquisition of K4me3 in GC 2000639 is observed. (c) K27ac sequence tag alignments predict the presence of a T allele at position chr7:27,228,085 while the reference (hg19) exhibits an A at this site. This site does not correspond to a known dbSNP. (d) Sanger sequencing and pyrosequencing validation of genotypes in input normal DNA, input tumor DNA and K27ac-enriched ChIP-seq DNA. The normal sample is homozygous for the A allele, while the cancer has a small T signal at this position (estimated allele frequency 10%). In contrast, K27ac-enriched DNA exhibits a high proportion of T alleles (96%). (e) TF site predictions by TFBIND for reference and somatically mutated alleles. LYF1, STAT and NF1 sites are predicted to be gained, while CEBP, NFKB and p53 sites are predicted to be lost. (f) Luciferase reporter assays measuring regulatory activity of wild-type and mutant alleles. DNA containing the mutant allele provides increased transcriptional activity (*P=1.1 × 10−4, Student’st-test). Experiments were performed in KATOIII GC cells, and replicated three times. Error bars were defined as s.e.m. (n=3). 15 , Supplementary Table 5 ). GCs exhibiting high expression of K4me3-marked genes exhibited higher M-stages ( P =0.033, Pearson’s χ 2 test; Supplementary Table 6 ; Supplementary Fig. 16 ), diffuse Lauren’s histology ( P =9.99 × 10 −5 , Pearson’s χ 2 test; Supplementary Table 6 ; Supplementary Fig. 16 ), and worse overall survival compared with GCs where these genes were lowly expressed ( Fig. 2j ; P =0.04, log-rank test). Multivariate Cox regression analysis revealed that the survival outcomes not independent of tumour stage ( P =0.74, Wald test). Genes driven by K4me3-marked promoters in GC may thus contribute to pathologic and clinical features of GC. Genomic features of cancer associated promoters When mapped against genomic occupancy data of 161 transcription factors (ENCODE consortium [39] ), cancer-associated promoters exhibited a generalized depletion of previously defined transcription factor binding sites (TFBSs) ( Fig. 3a , Supplementary Fig. 17 , Supplementary Table 7 ), but a significant enrichment in SUZ12 and EZH2 binding ( P =1.2 × 10 −24 and P =1.1 × 10 −4 for SUZ12 and EZH2, one-tailed Fisher’s exact test, Bonferroni corrected). SUZ12 and EZH2 are components of PRC2, an epigenetic regulator complex that targets key developmental genes in ESCs [40] . PRC2 is also involved in cancer progression [41] . In contrast, GC-associated predicted enhancers did not display SUZ12/EZH2 enrichment, but were associated with developmental regulators including forkhead (FOX), GATA family members and the FOS and JUN cell cycle regulators ( P <0.05, one-tailed Fisher’s exact test) ( Fig. 3b ). Figure 3: Binding site analysis of cancer-associated regulatory elements. ( a ) Frequency of ENCODE-defined TFBSs overlapping with cancer-associated promoters (gained and lost). Values are presented as the number of TFBS per 10 kb coverage. TFs were sorted according to their frequency in all K4me3-defined promoter sets. EZH2, SUZ12 and ZNF217 binding sites are enriched ( P <0.05, one-tailed Fisher’s exact test). The complete TF list is presented as Supplementary Fig. 17 and Supplementary Table 7 . ( b ) TFBS frequency in cancer-associated predicted enhancer regions. ( c ) Overlap analysis between ESC-defined univalent (K4me3 only, K27me3 only) or bivalent (K4me3 and K27me3) regions and GC promoters (all and cancer-associated) and GC-predicted enhancers (all and cancer-associated). Cancer-associated GC promoters exhibit an elevated proportion of bivalent regions, exceeding univalent regions ( P <2.2 × 10 −16 , one-tailed Fisher’s exact test). ( d ) Genome browser view of the ONECUT2 locus as a representative cancer-associated promoter overlapping with an ESC-defined bivalent region. ( e ) Box plot depicting changes in DNA methylation β-values in all promoters and cancer-associated promoters (gained or lost). P -values (Wilcoxon test) are: P =7 × 10 −48 (all promoters versus gained promoters); P =0.48 (all promoters versus lost promoters); P =5.37 × 10 −41 (gained promoters versus lost promoters). Full size image Several common themes were observed between GC-associated promoters and PRC2-targeted regions in ESCs. First, the SUZ12 sites overlapping with GC promoters were sourced from ESCs and embryonic carcinoma cells, and not other ENCODE cell types (for example, lymphoblastoid lines). Second, in ESCs, PRC2 binding is associated with bivalent/poised chromatin states (K4me3 and K27me3 positive) [42] , [43] , and similarly the GC promoters were enriched at regions exhibiting K4me3 and K27me3 bivalency in ESCs ( P <2.2 × 10 −16 , one-tailed Fisher’s exact test; Fig. 3c )—an example is shown for the homeobox gene ONECUT2 ( Fig. 3d ). Third, in ESCs, PRC2-targeted regions exhibit DNA methylation loss [44] . Using Illumina methylation arrays, we confirmed that GC-associated promoters also exhibited decreased DNA methylation levels relative to the overall population ( P =7.07 × 10 −48 , two-tailed Wilcoxon test) ( Fig. 3e ). Cancer-associated promoters in GC may thus be molecularly analogous to PRC2-targeted regions in stem cells. Germline variation in somatic regulatory elements We proceeded to explore genetic variation in GC-associated regulatory elements. Due to overall levels of sequence coverage in the Nano-ChIP-seq data being lower compared with conventional exome-sequencing studies [2] , [4] (mean coverage 29 × in combined K4me3, K4me1, K27ac and input data), we used MuTect, a recently described ultra-sensitive variant identification algorithm that provides accurate variation detection even in sequence data of lower coverage. Specifically, MuTect has been validated to be 90% accurate in sequence data of ≥20 × (ref. 45 ). While primarily designed to identify somatic variants, portions of the MuTect output can be adapted to also identify germline variants. Using MuTect, we interrogated 160 Mb of putative regulatory sequence with minimum 20 × sequence coverage in both GC and normal samples, and identified 249,930 single-nucleotide variants (SNVs) ( Supplementary Table 8 ). Of these, 99.9% of the SNVs (249,786) corresponded to previously reported germline SNPs (dbSNP137). The observation that almost all of the MuTect-identified SNVs are previously known germline SNPs suggests that despite lower sequence coverage levels, the Nano-ChIP-seq genetic variation data do not suffer from an excessive false-positive rate. Conversely, consistent with a low false-negative rate, the germline SNP detection rate in the Nano-ChIP-seq data (0.16%) is also comparable with that reported in the 1000 genomes project (0.12%) [46] . Among the germline SNPs, ~188,500 were heterozygous in at least one sample. We found that heterozygous SNPs mapping to regulatory elements could be divided into non-allele-biased and allele-biased sites. At non-biased sites, Nano-ChIP-seq sequence reads exhibited an equal proportion of reference and variant alleles. For example, GC 2000639 exhibited a cancer-associated promoter at the TNK2 gene locus ( Fig. 4a,b ). In normal DNA from this patient, this region was heterozygous for dbSNP rs7636635 ( Fig. 4c ), and similarly in the tumour, the K4me3-enriched reads were contributed by an equal proportion of reads bearing both reference and rs7636635 alleles ( Fig. 4c,d ). In contrast, allele-biased sites displayed Nano-ChIP-seq reads skewed towards one allele. This was observed in a cancer-associated promoter at the NUDT4 locus ( Fig. 4e,f ). Analysis of normal DNA from this patient confirmed heterozygosity for rs4761701 ( Fig. 4g ), but in tumours, the K4me3-enriched reads were primarily contributed by reads bearing the rs4761701 allele rather than the reference allele ( Fig. 4g,h ). Figure 4: Allele-specific regulatory elements associated with GC. ( a – d ) Non-allele biased and ( e – h ) allele-biased regulatory elements. ( a , b ) Genome browser view of TNK2 locus showing RNAseq and K4me3 tracks. ( b ) Close-up visualization of K4me3 sequence tags and SNPs. A comparable proportion of reference (C) and rs7636635 (T) SNPs are observed in K4me3-enriched sequence reads. ( c ) Genotyping of normal tissue confirms equivalent allele heterozygosity in normal tissues and K4me3-enriched sequence tags from tumours. ( d ) qPCR pyrosequencing confirms lack of K4me3 signal in normal tissue, and equal proportion of reference (C) and rs7636635 (T) allele K4me3-enriched sequence reads from tumours. Error bars are s.e.m. of qPCR signal ( n =3). ( e , f ) Genome browser view of NUDT4 locus showing RNAseq and K4me3 tracks. (f) Close-up visualization of K4me3 sequence tags and SNPs. A bias favoring a higher proportion of rs4761701 SNP (A) over the reference allele (G) is observed. ( g ) Genotyping of normal tissue confirms equivalent allele heterozygosity in normal tissues but a bias towards rs4761701 SNP (A) in K4me3 sequence tags from tumours. ( h ) qPCR pyrosequencing confirms minimal K4me3 signal in normal tissue, and an rs4761701 SNP-biased proportion of sequence tags over the reference allele in K4me3 signals from tumours. Error bars are s.e.m. of qPCR signal ( n =3). ( i ) Allele bias distribution across samples. Over- and underrepresentation of SNP tags in tumor tissues are marked in green and blue. ( j ) dbSNP sites mapping to altered regulatory regions. SNP sites are ordered following their chromosomal position ( x axis), and allele bias levels ( y axis). SNPs exhibiting allele bias (above blue horizontal line) and also predicted to affect protein binding based on RegulomeDB are marked in red. ( k , l ) Genome browser view of the KLK1 locus showing RNAseq and K4me3 tracks. ( l ) Close-up view of K4me3 sequence tags and SNPs. A bias favoring a higher proportion of the known eQTL SNP rs2659104 (G) over the reference allele (A) is observed. ( m ) qPCR pyrosequencing confirms minimal K4me3 signal in normal tissue, and rs2659104 SNP-biased proportions of sequence tags over the parental allele in K4me3 signals from tumours. Error bars are s.e.m. of qPCR signal ( n =3). Full size image We reasoned that the allele-biased sites in cancer samples might be caused by either loss of heterozygosity, or active enrichment of particular alleles for chromatin marks (allele-specific regulatory elements). To identify allele-specific regulatory elements associated with cancer, we overlapped heterozygous sites exhibiting allele bias (SNP overrepresentation of >30%; Fig. 4i ) with regions exhibiting chromatin mark alterations between GCs and normal tissues. We identified 714 heterozygous SNPs associated with chromatin mark differences (K4me3, K4me1, K27ac) between GC and normal samples—of these, 17.6% (126/714) exhibited an allele bias. Interestingly, this percentage is significantly greater than alleles associated with unchanged chromatin marks between GCs and normal samples (11.5%, 5471/47537; P =1 × 10 −6 , one-tailed Binomial test). Overall, these percentages are comparable to that reported in recent studies [47] , [48] . Of 126 candidate sites ( Fig. 4j ), we focused on 16 SNPs (13%) predicted by RegulomeDB, a database of human regulatory variants, to influence protein DNA binding (RegulomeDB score 1 or 2) [49] ( Table 1 ). Eleven of these 16 sites could be further validated by quantitative pyrosequencing (five sites could not be assayed due to PCR or sequencing failures), and of these 11, we confirmed the presence of allele bias in eight sites (73%) within Nano-ChIP-enriched reads but not in cancer and normal input DNAs, indicating that this bias is not due to loss of heterozygosity in the cancer tissues ( Supplementary Table 9 ). Four alleles corresponded to previously identified eQTLs ( Table 1 ), including the KLK1 gene that showed allelic bias for the eQTL dbSNP rs2659104 ( Fig. 4k–m ). These results highlight a potential role for allele-specific regulatory elements in controlling patterns of GC gene expression, as several genes associated with the allele-biased sites have been previously implicated in GC (for example, CLDN4 [50] , MTAP [51] , SERPINB5 [52] ). Table 1 RegulomeDB predictions for allele-biased germline variants in somatically altered regulatory elements. Full size table Somatic mutations in somatic regulatory elements Besides germline SNPs, we also identified 144 putative somatic mutations, representing genetic variations present in GCs but not in matched normal tissues. To validate these predicted somatic mutations, we performed Sanger sequencing of both tumour and matched normal genomic DNAs for 71 sites and validated 55 sites as being bona fide somatic mutations ( Supplementary Fig. 18 ), leading to an overall accuracy rate of 77%. Given the recognized sensitivity limitations of Sanger sequencing, it is likely that this figure represents a lower limit. Among the validated somatic mutations, we observed mutations associated with CDH10 , FAR2 and HOXA11 ( Fig. 5 , Supplementary Figs 19–21 ). Interestingly, both the CDH10 and FAR2 mutations exhibited allele bias in K4me3-enriched reads relative to input tumour DNAs, and also tumour-associated gene expression. Figure 5: Somatic regulatory mutations in GC. ( a ) Genome browser view of the HOXA locus. (top) RNAseq data. HOXA genes distal to (and including) HOXA11 are expressed in GC 2000639 in a cancer-specific fashion. (Bottom) K4me3 signals confirm an altered chromatin domain in this region. ( b ) Close-up view of the HOXA11 region. Cancer-specific acquisition of K4me3 in GC 2000639 is observed. ( c ) K27ac sequence tag alignments predict the presence of a T allele at position chr7:27,228,085 while the reference (hg19) exhibits an A at this site. This site does not correspond to a known dbSNP. ( d ) Sanger sequencing and pyrosequencing validation of genotypes in input normal DNA, input tumor DNA and K27ac-enriched ChIP-seq DNA. The normal sample is homozygous for the A allele, while the cancer has a small T signal at this position (estimated allele frequency 10%). In contrast, K27ac-enriched DNA exhibits a high proportion of T alleles (96%). ( e ) TF site predictions by TFBIND for reference and somatically mutated alleles. LYF1, STAT and NF1 sites are predicted to be gained, while CEBP, NFKB and p53 sites are predicted to be lost. ( f ) Luciferase reporter assays measuring regulatory activity of wild-type and mutant alleles. DNA containing the mutant allele provides increased transcriptional activity (* P =1.1 × 10 −4 , Student’s t -test). Experiments were performed in KATOIII GC cells, and replicated three times. Error bars were defined as s.e.m. ( n =3). Full size image We focused on the HOXA11 -associated A>T mutation, due to the involvement of HOXA11 in numerous cancers [53] , [54] . Five lines of evidence suggest that this somatic mutation is functional and not a bystander alteration. First, presence of this mutation in GC 2000639 was associated with K4me3 and K27ac promoter mark gain ( Fig. 5a–c ). Second, presence of this mutation was associated with upregulated HOXA11 locus RNA expression in GCs ( Fig. 5a ). Third, in the K27ac sequence reads, the T-mutant allele exhibited allele bias, being highly overrepresented (96%) relative to input tumour DNA where its somatic mutation allele frequency is ~10% or less ( Fig. 5c,d ). Fourth, presence of this mutation is predicted to alter TFBSs [55] ( Fig. 5e ). Fifth, in a luciferase reporter assay, genomic DNA fragments bearing the mutant T allele exhibited significantly greater transcriptional activity, compared with genomic DNA bearing the wild-type A allele ( P =1.1 × 10 −4 , Student’s t -test, Fig. 5f ). These results demonstrate that Nano-ChIP-seq can identify functional regulatory somatic mutations in GC, particularly when coupled with sensitive variant detection algorithms such as MuTect [45] . Regulatory elements are estimated to occupy 1.5–10% of the human genome [56] , and strongly influence development and disease [57] , [58] . However, locating these elements, and defining biological states regulating their activity, remains an important challenge. Here, we used Nano-ChIP-seq to perform a genome-wide survey of histone modifications and their associated regulatory elements in primary GCs. While our study should be considered a first-pass survey due to the limited number of GCs profiled, we made several notable observations that improve our overall understanding of gastric tumorigenesis. First, we characterized, for the first time, landscapes of promoters and predicted enhancer elements located in non-coding regions of the genome that are somatically altered in primary GCs. Second, we found that a large proportion of cancer-associated promoters were cryptic, suggesting that in GC, there is a widespread activation of non-canonical promoters resulting in altered transcriptional usage of 5′ exons. Third, we identified specific germline variants located within the somatically altered regulatory elements that exhibit allelic bias—such variants may highlight germline alleles that predispose normal gastric tissues to the development of GC. Finally, in the literature, only a handful of examples are known about potential regulatory mutations in cancer [59] , [60] . In a proof-of-concept, we demonstrate how the Nano-ChIP-seq data can be analysed to identify potential ‘driver’ somatic mutations in the HOXA11 non-coding region, which may cause the creation of new regulatory elements and influence transcriptional patterns. Such a strategy could be conceivably be extended and expanded in future to identify additional non-coding regulatory mutations in GC and other cancer types. We note that our study is not without limitations. For example, although previous studies have successfully used histone marks (particularly K4me1) to predict enhancers [25] , [30] , [31] , it is worth noting that while many enhancers exhibit these marks, the same marks could also be present in other regions that are not necessarily enhancers (for example, distal DNase I hypersensitive sites [61] ). In our study, technical validation of our enhancer prediction method benchmarking ENCODE histone mark data against known TFBSs yielded varying levels of enhancer prediction accuracy depending on cell line ( Supplementary Table 3 ). Importantly however, the overlap of each TFBS against our predicted enhancers remained highly significant ( P <1 × 10 −4 , assessed by random permutation, Supplementary Fig. 5 ). These results indicate that among the ~125 K enhancer predictions in our GC study, the number of true enhancers is probably smaller. The use of more sophisticated bioinformatic algorithms and/or additional secondary filters in future research should help to pinpoint more true enhancers. Another caveat is that although our pipeline has reasonable specificity for a proof-of-concept study (77%), the somatic mutation rate in the Nano-ChIP-seq data (0.9 mutations per Mb) is lower than somatic mutation rates reported in exome-sequencing studies of colon and rectal cancer, which are also gastrointestinal cancers (eight mutations per Mb [62] ). These differences could be due to several reasons including chromatin organization, as somatic mutation rates have recently been shown to negatively correlate with levels of euchromatin-associated histone modification (that is, K4me3, K27ac and K4me1) [63] . Alternatively, our lower sequence coverage levels, compared with cancer exome-sequencing studies, may have caused certain somatic mutations to be missed, particularly those occurring in subclonal tumour populations. These observations point the way for subsequent research. In the future, Nano-ChIP-seq could be expanded to other tumour types and even to smaller cell numbers, facilitating analysis of diagnostic biopsies and drug resistant clones [23] . From a translational perspective, our findings also suggest that cryptic promoters, and their associated non-canonical transcripts, could be conceivably exploited as biomarkers for cancer diagnostics. Tissue samples Primary patient samples were obtained from the SingHealth Tissue Repository, and collected with approvals from institutional research ethics review committees and signed patient informed consent. ‘Normal’ (that is, non-malignant) samples used in this study refer to samples harvested from the stomach, from sites distant from the tumour and exhibiting no visible evidence of tumour or intestinal metaplasia/dysplasia upon surgical assessment. Tumour samples were confirmed by cryosectioning to contain >40% tumour cells. Nano-ChIP-seq Fresh-frozen cancer and normal tissues were dissected using a razor blade in liquid nitrogen to obtain ~5-mg-sized pieces (~5 μl by apparent volume). Tissue pieces were fixed in 1% formaldehyde/TBSE buffer (20 mM Tris–HCl, 150 mM NaCl, 1 mM EDTA) for 10 min at room temperature. Fixation was stopped by addition of glycine to a final concentration of 125 mM. Tissues were washed three times with TBSE buffer, and transferred into Lysonator cartridges (SG Microlab Devices, Singapore). Tissues were dissociated at 4 KHz for 3 min, recovered into 1.5 ml microfuge tubes and centrifuged (5,000 r.p.m., 5 min). Dissociated tissue pellets were taken directly to the lysis step in the Nano-ChIP assay [23] . Dissociated tissues were lysed in 200 μl 1% SDS lysis buffer and divided into two 1.5 ml tubes for sonication (total 6 min, 30 s pulses with 30 s interval in ice-cold water bath) using a Bioruptor (Diagenode). Sonicated samples were diluted with 10 × volume of 0.01% SDS buffer and precleared with Dynal Magnetic beads (Invitrogen/Life Technologies). Chromatin solutions were centrifuged for 10 min at 10,000 r.p.m., and the supernatant was divided into five immunoprecipitation and input samples. For each tissue, ChIPs were performed overnight using the following antibodies at SDS and NaCl final concentrations: K4me3 (07–473, Millipore, 2 μl per ChIP, 0.1% SDS, 140 mM NaCl); K4me1 (ab8895, Abcam, 3 μl per ChIP, 0.2% SDS, 140 mM NaCl); K27ac (ab4729, Abcam, 2 μl per ChIP, 0.3% SDS, 140 mM NaCl); K36me3 (ab9050, Abcam, 1 μl per ChIP, 0.4% SDS, 280 mM NaCl); K27me3 (07–449, Millipore, 3 μl per ChIP, 0.2% SDS, 140 mM NaCl). ChIP beads were washed four times with 0.01% SDS buffer, then once with TE buffer and collected on a magnetic stand. Reverse cross-linking was performed with Pronase (Roche) at 42 °C for 2 h, then 68 °C for 6 h. After recovery of ChIP and input DNA by phenol–chlorform–isoamyl alcohol extraction and ethanol precipitation, whole-genome amplification was performed using the WGA4 kit (Sigma-Aldrich) and BpmI-WGA primers. Amplified DNAs were purified using PCR purification columns (Qiagen), digested with BpmI (New England Biolabs) and column-purified. BpmI digested WGA products were ligated to a second BpmI adaptor using T4 DNA ligase (New England Biolabs) and digested again by BpmI overnight to trim WGA primer regions and semi-random priming ends. Processed WGA products were quantified using a Quant-it Picogreen kit (Invitrogen). 15 ng of amplified DNA was used for each Illumina sequencing library construction (Illumina). Each library was sequenced on one lane of HiSeq2000 to obtain either 36- or 101-base single reads. Nano-ChIP-seq read mapping and peak calling Sequencing tags were mapped against the human reference genome (hg19) using Burrows-Wheeler Aligner software (version 0.7.0) and the ‘aln’ algorithm. Hundred and one base reads were trimmed by the first and last 10 bases to increase SNP call performance. Uniquely mapped tags were used for peak calling by CCAT version 3.0. Peak regions were filtered by a fold-above input cut-off of 8 for K4me3, K27ac, 5 for K4me3 and K36me3 and 1.5 for K27me3 marks. For K4me3 and K4me1 histone modifications, peak regions from all tissue samples were pooled, and overlapping peak regions were merged to create a total set of peak regions for that modification for promoter and enhancer analysis. Normal input versus cancer input CCAT3 region sets with the same fold-cut-off were used to remove potential amplified regions for K4me3 and K4me1 regions. To quantify peak heights, we analysed the ChIPseq data using Cufflinks (version 2.0.2) [64] . RPKM values were estimated for K4me3 and K27ac for promoter regions, K4me1 and K27ac for predicted enhancer regions. Batch effects were assessed using PCA and adjusted using ComBat [65] after log2 transformation of RPKM values. 3D-PCA plots were plotted using the ‘ rgl ’ package in R (version 2.15). Validation of enhancer predictions The performance of our enhancer predictions was independently validated using cell line data from the ENCODE consortium [32] . Specifically, CCAT [27] version 3.0 was used to detect peaks from K4me1 and K4me3 for cell lines HeLaS3 and K562. Statistically significant peaks (CCAT, FDR<0.05) were deemed as putative regulatory regions. To predict enhancers, we focused on regions enriched for K4me1 but excluding K4me3. Subsequently, we assessed sensitivity and specificity by comparing the enhancer predictions with binding sites of three different transcription factors (TFBS)—P300, CEBP and CTCF previously defined by ENCODE. We considered distal TFBSs located at least 2.5 Kb away from known 5’ ends of genes (as determined by GENCODE [66] version 19). Enhancer predictions were considered true if one of the aforementioned TFBS was located within 500 bp. To assess the significance of overlap between enhancer predictions and TFBS, we randomly assigned the same number of enhancer predictions and linked them to TFBS using the same criteria, running this procedure for 10,000 iterations. Identification of somatically altered regulatory elements Somatically altered promoter and predicted enhancer sets were identified using two methods—a ‘threshold’ method and a linear model approach. The final set of altered elements was generated by combining the results from both methods. ‘Threshold’ method K27ac ChIP-seq ComBat-adjusted RPKM values for all promoters (K4me3 marked) and predicted enhancers (K4me1 marked, but not overlapping with K4me3 peak regions) were filtered by (i) greater than twofold (absolute) change and (ii) greater than 0.5 (absolute) difference in mean values between five tumour and five normal samples. This was also performed for the K4me3 and K4me1 ChIP-seq data. Altered elements were identified from the union of regions obtained for K27ac and K4me3 analyses (promoters), or K27ac and K4me1 (predicted enhancers). Linear model method Box plots were plotted for the log2-transformed ChIP-seq data to assess the normality assumption, prior to applying an empirical Bayes linear model approach to obtain differentially altered regions between the tumour and normal samples ( Supplementary Fig. 6 ). After the model was fitted, assessment was also made to ensure P -value distributions were reasonable ( Supplementary Fig. 6 ). To obtain altered promoters and predicted enhancers, a P =0.05 threshold (empirical Bayes moderated statistical t -test) level of significance was taken. PCR validation of somatically altered elements Somatically altered elements detected by Nano-ChIP-seq were validated by qPCR. Nano-ChIPed and input DNAs from three GCs and matched normal controls were tested for 18 somatically altered elements (9 K27ac, 9 K4me3) by qPCR using a SYBR Green PCR kit (Life Technologies, USA). qPCR values from Nano-ChIPed DNAs were normalized against input DNA values. All qPCR reactions were performed in triplicate. Pearson’s correlation coefficients were computed, and P -values derived from Student’s t -test distribution. Primer sequences used are in Supplementary Table 10 . RNAseq RNAseq libraries were prepared using Illumina Tru-Seq RNA Sample Preparation v2 protocol, according to the manufacturer’s instructions. Libraries were validated with an Agilent Bioanalyzer (Agilent Technologies, Palo Alto, CA), diluted to 11 pM and applied to an Illumina flow cell using the Illumina Cluster Station. Sequencing was performed on an Illumina HiSeq2000 sequencer at the Duke-NUS Genome Biology Facility with the paired-end 76 bp read option. RNAseq analysis Reads were aligned to the human reference genome using TopHat v1.2 (ref. 67) [67] . Unmapped reads were then aligned to potential splice junctions that were either: (i) present in Ensembl 60 transcript annotations, or (ii) suggested by ‘expression islands’—that is, clusters of reads from transcripts that were not present in the annotations. Transcript abundances by FPKM (fragments per kilobase of transcript per million mapped reads) value were estimated using Cufflinks (version 1.0.0) without using reference transcripts. De novo assembled transcripts from the tumour/normal pairs were filtered against the RefSeq transcript database to identify non-RefSeq annotated regions. RefSeq TSS overlap analysis RefSeq and GENCODE transcripts were downloaded from the UCSC browser while ENSEMBL transcripts were queried using BioMart. Annotated TSSs were defined by extending transcript start positions by ±500 bases. Somatically altered K4me3 peak regions were compared against RefSeq TSS regions to determine overlaps. K4me3 regions with no overlap with RefSeq TSSs (±500 bases) were deemed non-RefSeq promoters (aka cryptic promoters). De novo assembly of RNAseq reads was performed by Cufflinks (version 1.0.0) without the reference transcript set. Non-RefSeq transcripts were defined by filtering the Cufflinks de novo exon output against the RefSeq exons (minimum 1-base overlap). This non-RefSeq transcript set was intersected against the cancer-associated K4me3 regions (minimum 1-base overlap, mean overlap 920 bp, median overlap 517 bp). Validation of cryptic promoters in GC cell lines Cryptic promoters observed in primary GCs were interrogated against K4me3 and K27ac Nano-ChIP-seq data from four GC cell lines (N87, YCC3, OCUM1 and SNU16), obtained from Yonsei Cancer Centre, Japanese Collection of Research Bioresources Cell Bank or the American Tissue Type Collection. Nano-ChIP-seq sequence reads from the cell lines were trimmed, mapped, filtered by mapped quality score (threshold of 10), and subjected to peak calling. To detect the presence of cryptic promoters in the cell lines, the cell line peaks were intersected with cryptic promoter regions using bedtools . Quantitative RT–PCR for transcript validation qPCR was performed using a SYBR Green PCR kit (Life technologies, USA). GAPDH was used as a control gene for normalization. All PCR reactions were performed in triplicate. Primers used are presented in Supplementary Table 10 . 5′ Rapid amplification of cDNA ends 5′ Rapid amplification of cDNA ends (5′ RACE) was performed using the 5′ RACE System for Rapid Amplification of cDNA Ends (version 2) kit (Invitrogen). One microgram of total RNA was used for each reverse transcription reaction with the Moloney Murine Leukemia Virus reverse transcriptase, and gene-specific primers for MET RefSeq exon 3 (5′-CTTCAGTGCAGGG-3′) or NKX6-3 RefSeq exon 1 (5′-GAAGGTAGGCTCCTC-3′). RNase H and RNase T1 were used to degrade the RNA, followed by the purification of first strand cDNAs with S.N.A.P. columns. Homopolymeric tailing of cDNAs were then used to create abridged anchor primer binding sites. Amplification of first strand cDNAs was performed using SuperTaq Plus Polymerase (Applied Biosystems) for 5′ RACE outer PCR with the abridged anchor primer, and gene-specific primers for MET exon 3 (5′-GGCTCCAGGGTCTTCACCTCCA-3′) and NKX6-3 exon 1 (5′-CCAGGCTGAGCACCGAGAAGGC-3′). Subsequently, 5′ RACE inner nested PCR was performed with the abridged universal amplification primer (AUAP), and the gene-specific primers for MET exon 3 (same as outer 5′ PCR) and NKX6-3 exon 1 (5′-GCTTGCGCAGCAGCAGGCGGAT-3′). Gel electrophoresis was performed, and PCR bands of interest were excised for cloning with a TOPO TA Cloning Kit with pCR 4-TOPO vectors (Invitrogen). A minimum of five independent colonies were isolated, and the purified plasmid DNA were sequenced bi-directionally on an ABI 3730 automated sequencer (Applied Biosystems). Western blotting GC cells were harvested in lysis buffer (10 mM Tris–HCl (pH7.5), 150 mM NaCl, 1% Triton X-114) in the presence of protease inhibitors for 10 min on ice and centrifuged at 9000, r.p.m. for 15 min. Supernatants were incubated at 95 °C for 10 min before being processed for gel electrophoresis. Western blotting was performed with the following antibodies and dilutions: Met (C-12) (1:250; sc-10 Santa Cruz) and β-actin (1:2,000; Proteintech). Experiments were repeated in triplicate. Microarray analysis GC (200) and 100 matched normal gastric samples profiled on Affymetrix Human Genome U133 Plus 2.0 Genechip arrays were analysed (GSE 15459). Data pre-processing was carried out using the ‘ affyPLM’ R package (v 2.15). Outliers were excluded, giving a total of 185 GC and 89 normal samples available for downstream analyses. Differential expression analysis between GC samples was performed using the ‘limma’ R package (v 2.15). Genes with FDR <0.05 were considered to be differentially expressed. Genes used for differential expression analysis were those emerging from the GREAT (v 2.02) analysis performed on the list of non-RefSeq transcripts from RNAseq analysis. For survival analysis, the GC samples were clustered using a K-medoids approach aimed at finding K that minimizes the silhouette width. To assess correlation of different GC groups with clinicopathological factors, a mosaic plot was plotted for categorical variables while a linear regression approach was employed for continuous variables. Significance (that is, P <0.05) of the correlation was determined by a Pearson χ 2 test or a t -test accordingly. Kaplan–Meier survival analysis was employed with overall survival as the outcome metric. The log-rank test was used to assess the significance of the Kaplan–Meier analysis. Univariate and multivariate analyses were performed using Cox regression. TFBSs analysis (ENCODE) ENCODE ChIP-seq TFBS data sets (TxnFacChIP V3—Transcription Factor ChIP-seq Clusters V3, 161 targets, 189 antibodies) were obtained from the UCSC browser. Overlaps against cancer-associated promoters and predicted enhancers (or all promoters and predicted enhancers) were counted for each TF. TF site counts were divided by the base coverage length of each corresponding promoter, enhancer or total set to calculate the TF site frequency per 10 kb coverage. DNA methylation profiling Illumina HumanMethylation450 (HM450) Infinium DNA methylation arrays were used to assay DNA methylation levels between the gastric tumour/normal pairs. Methylation β-values were calculated and background corrected using the methylumi package in R package version 2.4.0. Normalization was performed using the BMIQ method (wateRmelon package in R) [68] . Probes containing SNPs and repeats were removed. In addition, probes on the X and Y chromosomes were also removed. Control groups used included all 21,692 promoter regions. For each group (control, gain and loss), we identified HM450 probes overlapping with the promoter regions (135606, 2268, 963 probes for all, cancer-gained and cancer-lost, respectively). Probes with a detection P -value >0.05 (based on Illumina GenomeStudio P -value definition) were excluded. Probes that had an average change in DNA methylation, between the tumour and normal pairs, of at least 0.2-β (in either direction) were selected and plotted. A two-sample Wilcoxon test was performed. Single-nucleotide variation detection The sequencing data were pre-processed according to the best practices workflow in Genome Analysis Toolkit (GATK version 2.6) [69] . Specifically, samtools [70] was used to remove PCR duplicates. The remaining sequences were corrected for misalignments due to the presence of indels followed by base quality score recalibration. SNVs in each GC/normal pair were called using MuTect [45] . We used SNV attributes reported by MuTect to classify the SNVs as either dbSNP sites or potential somatic mutations. dbSNP sites have the following criteria: (i) it is a known dbSNP site, (ii) the site is powered to detect a mutation (a.k.a. covered site), (iii) the variant is supported by at least 20 × reads in GC and normal, and (iv) it passes the variant filters implemented in MuTect. Somatic mutations were identified using the following criteria: (i) it is a novel non-dbSNP variant, (ii) the alternate allele fraction in tumour is greater than 0.3 at a covered site, or 0.5 at uncovered sites, (iii) the site coverage has at least 20 reads in GC and normal, (iv) there is no mutant allele at the uncovered site in normal tissue. Besides MuTect, we also selected for Sanger validation somatic mutations identified using CLC Genomics Workbench (CLC Bio). Sanger sequencing to validate the somatic mutations were performed as follows: 15 ng of input-WGAed DNA from GCs and normal pairs were amplified in a 20 μl PCR reaction mixtures containing 10 μl of GoTaq hot start Taq colourless master mix (M5133, Promega) and 0.3 μM of primers. PCR conditions were: 95 °C for 2 min, followed by 35 cycles of 95 °C for 30 s; 58 °C for 30 s; 72 °C for 30 s and a final extension at 72 °C for 5 min. PCR products were purified by Exonuclease I (M0293L, New England Biolabs)–Thermosensitive Shrimp Alkaline Phosphatase (M9910, Promega) treatment. Purified PCR products were sequenced in both forward and reverse directions by using BigDyeTerminator v3.1 Cycle Sequencing Kit (Life Technologies). Purified pellets were dissolved in Hi-Di Formamide (4311320, Life Technologies) and analysed on a ABI PRISM 3730 Genetic Analyser (3730S, Life Technologies). Chromatograms were analysed by SeqScape V2.5 and manual review. Detection of allele bias We determined the alternate allele fraction at each site by computing alternate allele frequencies. Homozygous dbSNP sites showing an average alternate allele fraction greater than 0.9 in GC/normal pair were excluded. We focused on heterozygous sites showing an alternate allele fraction difference greater than 0.3 in a GC/normal pair (that is, allele bias). Allele-biased sites mapping to regions exhibiting cancer-associated chromatin mark alterations were assessed for functional impact using RegulomeDB [49] . For RegulomeDB hits, we also confirmed by quantitative pyrosequencing a lack of allele bias in input DNA populations. Quantitative pyrosequencing and TF site prediction Pyrosequencing was performed on a PyroMark Q24 (Qiagen). Results were analysed with PyroMark software for allele quantification. For ChIP–qPCR pyrosequencing, PCR primers were used for both real-time PCR quantification of ChIP DNA and allele quantification by pyroseqeuncing with WGA-amplified DNAs as a template. Quantification results and allele representations were combined to estimate the fraction of two alleles in the ChIP signal. Binding site predictions were performed using the TFBIND [55] ( http://tfbind.hgc.jp/ ). Luciferase assay Luciferase reporter assays were performed using Promega pGL3 (firefly luciferase) and pRLSV40 (Renilla luciferase) plasmids. The FOS gene promoter was amplified by PCR from human genomic DNA with BglII–HindIII linker primer, and ligated into the pGL3–BASIC plasmid. HOXA11 -associated fragments (~350 bp) containing either wild-type or mutated alleles were amplified from ChIP–WGA DNA with BglII linker primers, and cloned upstream of the FOS promoter. Insert directions and allele identities were confirmed by Sanger sequencing. KATO-III GC cells were seeded at 1 × 10 6 cells per 24-well plate, transfected with the pGL3 reporter or derivatives (100 ng per well), and pRLSV40 (20 ng per well) using Lipofectamine 2000 (Invitrogen). Cells were harvested 42 h post transfection, lysed in PLB buffer provided by the Dual-Luciferase Kit (Promega) and luciferase activity was measured. Reading of firefly luciferase activity was divided by renilla luciferase activity to normalize transfection efficiencies. Accession codes: Data for this manuscript has been deposited under GSE accession number GSE51776 How to cite this article: Muratani, M. et al. Nanoscale chromatin profiling of gastric adenocarcinoma reveals cancer-associated cryptic promoters and somatically acquired regulatory elements. Nat. Commun. 5:4361 doi: 10.1038/ncomms5361 (2014).